Interstitial oxygen as a source ofp-type conductivity in hexagonal manganites Hexagonal manganites, h- R MnO 3 ( R =Sc, Y, Ho–Lu), have been intensively studied for their multiferroic properties, magnetoelectric coupling, topological defects and electrically conducting domain walls. Although point defects strongly affect the conductivity of transition metal oxides, the defect chemistry of h- R MnO 3 has received little attention. We use a combination of experiments and first principles electronic structure calculations to elucidate the effect of interstitial oxygen anions, O i , on the electrical and structural properties of h-YMnO 3 . Enthalpy stabilized interstitial oxygen anions are shown to be the main source of p -type electronic conductivity, without reducing the spontaneous ferroelectric polarization. A low energy barrier interstitialcy mechanism is inferred from Density Functional Theory calculations to be the microscopic migration path of O i . Since the O i content governs the concentration of charge carrier holes, controlling the thermal and atmospheric history provides a simple and fully reversible way of tuning the electrical properties of h- R MnO 3 . Point defects are imperative to the functional properties of oxides used in electrochemical devices like solid oxide fuel cells, batteries and memristors [1] , [2] , [3] . In contrast, point defects in general have a detrimental effect on physical properties of oxides for electronics, such as for example fatigue and domain wall pinning in ferroelectrics [4] . As components are made smaller, the available length for point defects in materials to diffuse is made shorter. This reduces the time required for the point defect to diffuse through the samples compared with bulk materials, where they effectively freeze in [5] . Understanding point defects in functional oxides thus becomes ever more important with decreasing component dimensions [6] , [7] . Rare earth ternary manganites with R MnO 3 stoichiometry are stable in the hexagonal manganite structure with space group P 6 3 cm (185) for R =Sc, Y and Ho–Lu. The structure consists of layers of five-coordinated Mn 3+ corner-sharing trigonal bipyramids separated by layers of Y 3+ in the ab -plane. The MnO 5 bipyramids are tilted in a pattern of trimers, while the Y 3+ are displaced in opposite directions along the polar c -axis [8] . A subtle shift of the trigonal bipyramid layer with respect to the Y 3+ layer, caused by an improper ferroelectric transition at 1,250 K, is the origin of the ferroelectric polarization [9] . The Mn 3+ sublattice has a frustrated non-collinear antiferromagnetic order on a trigonal lattice, with a Néel temperature of 75 K (ref. 10 ). Compared with the ternary ABO 3 perovskite oxides, the defect chemistry of h- R MnO 3 has received little attention. Oxygen vacancies in YMnO 3 have been studied [11] , [12] , [13] , and large oxygen excess has been reported for h- R MnO 3+ δ ( R =Y, Dy) with δ up to 0.35 for R =Dy [14] . High levels of excess oxygen can cause development of secondary oxidized phases, which are easily detected experimentally [15] . However, structural effects, energetics and kinetics of point defects in low concentrations have not been addressed. Excess oxygen is well known in perovskite manganites such as LaMnO 3+ δ . Since the perovskite structure is too close-packed for interstitial oxygen anions, excess oxygen is accommodated by cation vacancies; La 1− δ /3 Mn 1− δ /3 O 3 (ref. 16 ). Oxidation of perovskite LaMnO 3 thus requires cation diffusion, which demands higher temperatures than anion diffusion. Diffusion of oxygen in bulk YMnO 3 has been observed below 200 °C (ref. 14 ), making cation vacancy compensation highly unlikely. The layered h- R MnO 3 structure is however ∼ 11% less dense than the corresponding orthorhombic perovskite structure, suggesting the possibility of interstitial oxygen. This is further supported by the observation that crystallization, which requires cation diffusion, of amorphous YMnO 3 only occurs above 800 °C (ref. 17 ). Here we investigate how excess oxygen in the form of highly mobile interstitial anions is accommodated in the hexagonal manganite structure, and demonstrate that this enthalpy stabilized point defect gives rise to the observed p -type conductivity in YMnO 3 . This shows the importance of controlling the material’s thermo-atmospheric history and opens a new avenue for tuning the physical properties of hexagonal manganites. Oxygen stoichiometry and electrical conductivity First we consider the effect of thermal and atmospheric history on the conductivity and oxygen stoichiometry of the prototypical hexagonal manganite YMnO 3 . Thermoelectric power for a porous polycrystalline YMnO 3 bar was measured in O 2 and N 2 atmosphere, Fig. 1a . The Seebeck coefficient is positive for all temperatures in O 2 atmosphere, implying that p -type electronic conduction dominates, and a maximum is observed at 300 °C. In N 2 atmosphere, the Seebeck coefficient is negative, implying conduction by electrons as majority charge carriers. The DC electrical conductivity of YMnO 3 in O 2 increases exponentially on heating from 100 °C, as expected for a semiconducting oxide. However, the conductivity goes through a maximum value at 270 °C, then decreases and stays relatively constant up to 420 °C, from which the conductivity again increases exponentially. In N 2 atmosphere, the DC conductivity follows an exponential trend on heating, as expected for a semiconductor. 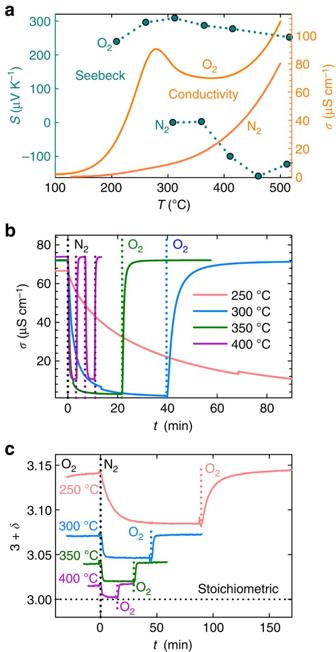Figure 1:p-type conductivity and excess oxygen. (a) Seebeck coefficient,S, and DC electrical conductivity,σ, in O2and N2atmosphere of a porous polycrystal of YMnO3, as a function of temperature,T. (b) DC electrical conductivity as a function of time,t, of a porous polycrystal upon switching atmosphere (indicated by dotted lines) between flowing O2and N2. The atmosphere is switched twice between O2and N2at 400 °C. (c) Oxygen stoichiometry, 3+δ, as a function of time,t, upon switching atmosphere measured by thermogravimetry for YMnO3nanoparticles (dXRD=49±4 nm). Figure 1: p -type conductivity and excess oxygen. ( a ) Seebeck coefficient, S , and DC electrical conductivity, σ , in O 2 and N 2 atmosphere of a porous polycrystal of YMnO 3 , as a function of temperature, T . ( b ) DC electrical conductivity as a function of time, t , of a porous polycrystal upon switching atmosphere (indicated by dotted lines) between flowing O 2 and N 2 . The atmosphere is switched twice between O 2 and N 2 at 400 °C. ( c ) Oxygen stoichiometry, 3+ δ , as a function of time, t , upon switching atmosphere measured by thermogravimetry for YMnO 3 nanoparticles ( d XRD =49±4 nm). Full size image The observations in Fig. 1a is consistent with the chemical defect reaction: where is interstitial O 2− , and and depicts Mn 3+ and Mn 4+ on Mn lattice sites, respectively. Tetravalent Mn in oxidized YMnO 3 is Mn with localized electron holes: . Holes as the majority charge carrier is consistent with the positive sign of the Seebeck coefficient. The mobility of negatively charged interstitial O 2− is expected to be orders of magnitude smaller than for holes, and this is addressed further below. The peculiar thermal evolution of the electrical conductivity can be explained from the maximum oxygen stoichiometry observed at about 250 °C (ref. 14 ), which coincides with a maximum in electrical conductivity. The deviation in conductivity from the exponential behaviour of a semiconductor stems from the different temperature dependence of the concentration and mobility of holes. While the mobility of holes increases with temperature, this is counterbalanced by the loss of oxygen and charge compensating holes, above 250 °C, as we will show further below. The atypical thermal evolution of the electrical properties of YMnO 3 in this temperature range has previously been attributed to the filling of oxygen vacancies [18] , [19] , [20] , but charge compensating electrons would give a negative Seebeck coefficient. DC conductivity measurements were then performed on isothermal change of atmospheres between O 2 and N 2 . When the partial pressure of oxygen, p O 2 , is reduced by switching from O 2 to N 2 atmosphere, the oxygen excess decreases according to equation (1) and a relaxation towards a lower conductivity is observed in Fig. 1b . The initial conductivity is regained after changing the atmosphere back to O 2 , demonstrating the reversibility of reaction (1). The regained conductivity is similar for all isotherms, owing to the opposing effects of decreasing charge carrier mobility and increasing concentration as the temperature is reduced. The relaxation time before equilibrium is reached is highly temperature dependent, as expected for diffusion of oxygen into the lattice. AC conductivity measurements were performed on samples annealed in flowing O 2 and N 2 , respectively, before measurement ( Supplementary Fig. 1 ). The conductivity of the O 2 annealed sample shows the characteristic maximum at 280 °C on heating, resembling the maximum observed in Fig. 1a . The conductivity measured on cooling is lower compared with the initial heating cycle reflecting the loss of O i that occurred at higher temperatures. The N 2 annealed sample exhibits a smooth increase of the conductivity with temperature. Subsequent cooling leads to higher conductivity in accordance with the reversibility of the O i incorporation process. The reversibility of reaction (1) is also evidenced by the oxygen stoichiometry when switching between O 2 and N 2 atmospheres, Fig. 1c . As the length scale of the system is imperative to diffusion controlled processes [5] , nanoparticles with an average crystallite size of d XRD =49±4 nm (ref. 17 ) were chosen for studying thermogravimetric relaxation on switching atmosphere at a shorter time-scale than in bulk material. With increasing temperature the oxygen stoichiometry equilibrates faster. The rapid change in oxygen stoichiometry in YMnO 3 nanoparticles illustrates the increasing importance of thermal and atmospheric history with decreasing system size. The isothermal response of the electrical conductivity ( Fig. 1b ) and the oxygen stoichiometry ( Fig. 1c ) on change in p O 2 is explained by reaction (1): oxygen hyperstoichiometry governs the electrical conductivity of h- R MnO 3+ δ . Position of interstitial oxygen and structural effects The low temperature at which YMnO 3 exchanges oxygen with the atmosphere makes cation vacancies and diffusion unrealistic, and the positive Seebeck coefficient from mobile holes points to interstitial oxygen anions, O i , as the dominating point defect. High-temperature X-ray diffraction measurements of nanocrystalline YMnO 3 show that interstitial oxygen is incorporated into the lattice, causing anisotropic chemical expansion ( Supplementary Fig. 2 ). We now turn our attention to the position of interstitial oxygen in YMnO 3 . Potential energy surfaces (PES) were determined by mapping the energy landscape of the O i position in several lattice planes by static Density Functional Theory (DFT) calculations (See details in Supplementary Fig. 3 and Supplementary Note 1 ). For illustration, the PES of O i in the (002) ( a ) and ( 3 / 2 00) ( b ) planes are included in Fig. 2 along wth a unit cell with the corresponding lattice planes ( d ). The relative energy of O i along the grey line in Fig. 2b is shown in Fig. 2c . The most stable positions of O i was found to be between three Mn in the Mn–O planes at z=0 and 1 / 2 , resulting in six equivalent possible sites for O i in the P 6 3 cm unit cell, ( 1 / 3 , 1 / 3 , 0), ( 2 / 3 , 0, 0), (0, 2 / 3 , 0), ( 2 / 3 , 2 / 3 , 1 / 2 ), ( 1 / 3 , 0, 1 / 2 ) and (0, 1 / 3 , 1 / 2 ), as illustrated by green circles in panels a and b . 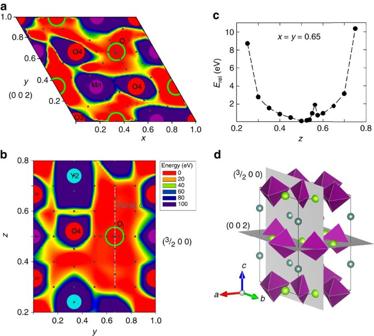Figure 2: Position of interstitial oxygen. Potential energy surfaces (PES) showing the energy landscape for the position of interstitial oxygen in a neutral YMnO3unit cell in (a) the (002) plane and (b) the (3/200) plane. (c) Relative energy along thezdirection forx=y=0.65 indicated by a light grey line in panelb. The anomaly atz=0.56 stems from that the PES mapping was done with static calculations. (d) Crystal structure of YMnO3showing purple MnO5polyhedra, turquoise Y atoms, and green spheres marking the six equivalent stable positions for Oiin the unit cell along with the two crystal planes in (a),(b). Figure 2: Position of interstitial oxygen. Potential energy surfaces (PES) showing the energy landscape for the position of interstitial oxygen in a neutral YMnO 3 unit cell in ( a ) the (002) plane and ( b ) the ( 3 / 2 00) plane. ( c ) Relative energy along the z direction for x = y =0.65 indicated by a light grey line in panel b . The anomaly at z =0.56 stems from that the PES mapping was done with static calculations. ( d ) Crystal structure of YMnO 3 showing purple MnO 5 polyhedra, turquoise Y atoms, and green spheres marking the six equivalent stable positions for O i in the unit cell along with the two crystal planes in ( a ),( b ). Full size image Experimental observations of a maximum δ of ∼ 0.35 (refs 14 , 15 ) can be rationalized from our DFT simulations. If two out of the six possible stable interstitial sites in the unit cell are occupied, a hypothetical fully oxidized structure of YMnO 3 would have a chemical formula of YMnO 3.33 or Y 3 Mn 3 O 10 . This will result in one O i and two out of three oxidized Mn in each Mn–O layer of the 30 atom unit cell. Accommodation of more than two O i per unit cell would require charge compensation across layers or further oxidation of Mn 4+ to Mn 5+ within the same layer. The in-plane distances between O i and Mn after structural relaxation depicted in Fig. 3a,b show that there are two shorter and one longer Mn–O i bond. O i is displaced towards two d 3 Mn 4+ ions (with a calculated magnetic moment of 3.06 μ B ), and away from one d 4 Mn 3+ ion (3.74 μ B ). The localization of holes on the two oxidized Mn ions gives three possible configurations of O i and its three surrounding Mn ions. The most stable positions of O i are triple wells due to asymmetric electrostatic attraction: O i with formal charge −2 has shorter bonds to the two Mn 4+ than to the single Mn 3+ . Details and discussion about the energetic asymmetry of this triple well and the effect of O i on the magnetism can be found in Supplementary Figs 4 and 5 and Supplementary Note 2 . 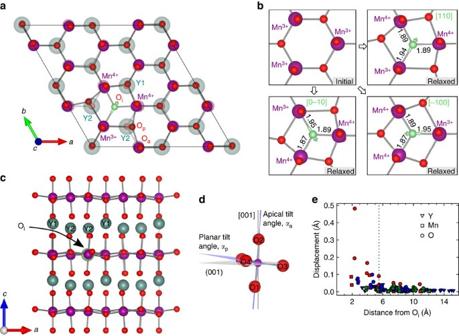Figure 3: Structural distortions and screening length. (a) Relaxed geometry of the (002) plane of a 2 × 2 × 1 supercell of YMnO3with the perfect structure faded in the background for comparison. Y atoms above the (002) Mn–O plane are projected onto the plane. (b) Unrelaxed structure in upper left panel compared with relaxed structures around Oiin the three triple-well positions around the2/3,2/3,1/2position. The green arrows on Oiindicate the displacement towards the two Mn4+. Bond lengths between Oiand Mn are given in Å. (c) YMnO3with Oi(green sphere in the (002) Mn–O layer) viewed along theb-direction. (d) Apical and planar tilting angles of the trigonal bipyramids. O1 and O2; and O3 and O4 being apical and planar oxygens, respectively. (e) Displacements of ions with respect to the perfect structure as a function of distance from Oi. The red symbols represent atoms in the same Mn–O layer as Oiis positioned, the blue symbols represent the apical oxygens and the yttrium atoms closest to the Mn–O layer with Oi, and the green symbols show atoms in the adjacent Mn–O layers. The structural screening length is indicated by a vertical dotted line. Figure 3: Structural distortions and screening length. ( a ) Relaxed geometry of the (002) plane of a 2 × 2 × 1 supercell of YMnO 3 with the perfect structure faded in the background for comparison. Y atoms above the (002) Mn–O plane are projected onto the plane. ( b ) Unrelaxed structure in upper left panel compared with relaxed structures around O i in the three triple-well positions around the 2 / 3 , 2 / 3 , 1 / 2 position. The green arrows on O i indicate the displacement towards the two Mn 4+ . Bond lengths between O i and Mn are given in Å. ( c ) YMnO 3 with O i (green sphere in the (002) Mn–O layer) viewed along the b -direction. ( d ) Apical and planar tilting angles of the trigonal bipyramids. O1 and O2; and O3 and O4 being apical and planar oxygens, respectively. ( e ) Displacements of ions with respect to the perfect structure as a function of distance from O i . The red symbols represent atoms in the same Mn–O layer as O i is positioned, the blue symbols represent the apical oxygens and the yttrium atoms closest to the Mn–O layer with O i , and the green symbols show atoms in the adjacent Mn–O layers. The structural screening length is indicated by a vertical dotted line. Full size image Localization of holes on Mn, and the resulting p -type polaronic conduction, stems from electrostatic attraction between positive holes and negative interstitial anions. In contrast, hole doping by substituting Y 3+ with Ca 2+ gives holes in Bloch states, while electron doping by Zr 4+ for Y 3+ substitution gives a polaronic state [21] . The energy barrier for moving the holes associated with O i between different Mn 4+ pairs is 0.29 eV from nudged-elastic band (NEB) calculations (See details in Supplementary Fig. 6 and Supplementary Note 3 ). Our calculated energy barrier is lower than the reported activation energy of 0.38–0.50 eV for polaron hopping in YMnO 3 (refs 22 , 23 , 24 ). Interstitial oxygen causes only subtle local structural distortions, as evident from the excerpt of the (002) plane of YMnO 3 in Fig. 3a . The relaxed atomic positions are shown in the foreground, while the atoms in a perfect crystal are included in faded colours in the background for comparison. The Y sublattice is virtually unaffected by the introduction of O i in the Mn–O layer, as shown in Fig. 3c . The local displacements of ions occur mainly within the same layer of trigonal MnO 5 bipyramids as O i is situated, and the distortions decrease rapidly with increasing distance from O i . The apical tilting angle, defined in Fig. 3d , of the three bipyramids surrounding O i is reduced from 8.7° in the perfect crystal to 6.4° for Mn 4+ bipyramids and 4.7° for Mn 3+ bipyramids, respectively. The local structural distortions caused by the introduction of O i can be quantified by the displacements of ions relative to the perfect P 6 3 cm structure as a function of the distance from the O i , as illustrated in Fig. 3e . Displacements of Mn and planar oxygen closest to O i are substantial, apical oxygen in the nearest bipyramids are also displaced, while Y even close to O i are less affected. The structural screening length of the O i point defect is defined here as the distance away from O i where the displacement is less than 0.1 Å relative to the perfect structure. A structural screening length can thus be estimated to 5.5 Å, corresponding to the second coordination shell of O i , and is shown by a dotted line in Fig. 3e . Local charge compensation of O i by two Mn 4+ and polyhedral tilting mitigates the effect of O i on the lattice. The short structural screening length implies that direct experimental detection of O i is challenging. The calculations also show that the non-collinear triangular magnetic order is only subtly affected by O i ( Supplementary Fig. 5 ). At the relevant temperatures for O i transport, the material is paramagnetic and the properties are therefore not expected to be significantly affected by magnetic order. The relaxed structure is not affected by substituting the true non-collinear magnetic ground state structure with a synthetic collinear magnetic order. Energetics of O i An essential thermodynamic quantity for point defects is the energy of formation. Using the formalism of Zhang et al . [25] for neutral cells we can define the energy of formation, E f , for interstitial oxygen as: where and are the total energies of oxidized and stoichiometric YMnO 3 , respectively, and μ O is the chemical potential of oxygen. The formation energy for O i in YMnO 3 as a function of the chemical potential of oxygen is shown in Fig. 4a (See Supplementary Fig. 7 and Supplementary Methods for details on the thermodynamic stability region for bulk YMnO 3 ). For , corresponding to air, the chemical potential of oxygen yields a negative formation energy at temperatures up to ∼ 900 °C, which is well above the temperature were O i becomes entropy destabilized, as seen from the experimental measurements in Fig. 1 . However, it must be pointed out that the formation enthalpy for O i is calculated in the dilute limit, while a finite concentration of O i is necessary to detect mass changes by thermogravimetry. The consumption of the gaseous species O 2 (g) in reaction (1) means that the entropy of this reaction is negative, hence the entropy contribution to the Gibbs free energy of (1) is positive. Given the negative enthalpy of reaction (1) from DFT, the Gibbs’ free energy of (1) becomes less negative with increasing temperature, gradually shifting (1) towards the left hand side where O i leaves the lattice to form O 2 molecules. The equilibrium concentration of O i hence decreases with increasing temperature, in line with the results in Fig. 1 , but in contrast to entropy stabilized oxygen vacancies which have a positive enthalpy of formation under conditions where the oxide is stable. In analogy to brownmillerite AB 2 O 5 and perovskite ABO 3 , O i in YMnO 3 could be considered filled oxygen vacancies in the hypothetical compound Y 3 Mn 3 O 10 . With Y 3 Mn 3 O 10 as the reference state, vacant O i sites would be oxygen vacancies, and thus conform to conventional point defect thermodynamics with positive enthalpies and entropies of formation. We note that the enthalpy of formation for O i is expected to decrease progressively with increasing oxygen excess δ due to O i –O i repulsion and a gradual loss of the driving force for oxidation. 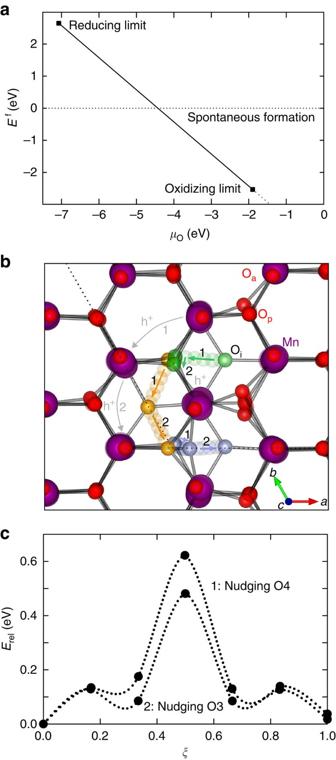Figure 4: Energetics and kinetics. (a) Defect formation energy of Oiin a 2x2x1 supercell of YMnO3as a function of chemical potential of oxygen. (b) Subsequent migration paths of Oi(green, then yellow and finally blue) through an interstitialcy mechanism nudging first a planar lattice oxygen at an O4 site (path 1) and then a planar lattice oxygen at an O3 site (path 2). The hopping of holes (h+) between Mn sites are shown by grey arrows. (c) The migration energy barriers for path 1 (nudging an O4) and path 2 (nudging an O3) as functions of the relative reaction coordinate,ξ. Figure 4: Energetics and kinetics. ( a ) Defect formation energy of O i in a 2x2x1 supercell of YMnO 3 as a function of chemical potential of oxygen. ( b ) Subsequent migration paths of O i (green, then yellow and finally blue) through an interstitialcy mechanism nudging first a planar lattice oxygen at an O4 site (path 1) and then a planar lattice oxygen at an O3 site (path 2). The hopping of holes (h + ) between Mn sites are shown by grey arrows. ( c ) The migration energy barriers for path 1 (nudging an O4) and path 2 (nudging an O3) as functions of the relative reaction coordinate, ξ . Full size image Migration of O i To investigate the ionic mobility of interstitial oxygen, migration paths for O i between two stable positions were investigated by NEB calculations. Simple interstitial migration, with a calculated energy barrier of almost 6 eV ( Supplementary Fig. 8a ), is not likely to occur. In the interstitialcy mechanism, O i pushes an adjacent planar oxygen into a neighbouring interstitial site, subsequently taking up a regular planar oxygen lattice position itself. The maximum energy along the minimum energy path is found when the distance between O i and planar lattice oxygen goes through a minimum. When O i nudges a regular oxygen at an O3 site, ( Fig. 4b ) an energy barrier of 0.48 eV was found ( Fig. 4c ). A similar mechanism where O i nudges a regular oxygen at an O4 site resulted in a higher energy barrier of 0.62 eV (See Supplementary Fig. 8b,c for effect of magnetic order and Hubbard U ). This is explained by Y1 being closer to the moving O3 (which is a trimerization centre) and O i in path 2 compared with the corresponding distance between Y2 and the moving O4 and O i in path 1 ( Fig. 4b ) (See Supplementary Fig. 8e and f for illustration of bond lengths). Migration through path 2 will therefore be aided by Y1 bonding to the two moving oxygen atoms, which is supported by the electronic density of states in Fig. 5d . An energy barrier was also estimated from the experimental TGA data by plotting time to oxidation as a function of annealing time in O 2 atmosphere, as shown in Supplementary Figure 8d . The Arrhenius-type relation gave an energy barrier of 0.55±0.21 eV, in agreement with our DFT calculated values. For comparison, oxygen transport through vacancy diffusion in ABO 3 perovskites has an energy barrier in the range of 0.5–2.8 eV (ref. 26 ). See Supplementary Note 4 for more details about the migration barriers. 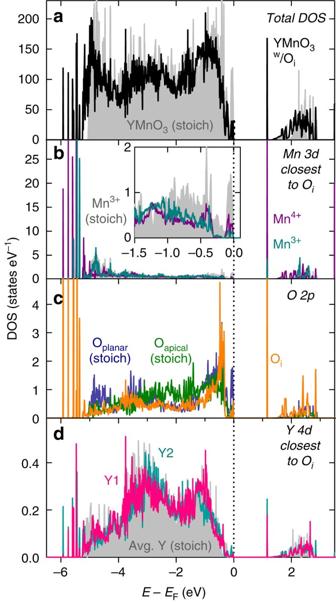Figure 5: Electronic structure. (a) Total electronic density of states (DOS) for a perfect 120 atom YMnO3cell and a 121 atom cell of YMnO3with one Oi(YMnO3.04). (b) Atomic DOS showing thedstates for Mn3+and Mn4+coordinating Oicompared with Mn3+dstates in a stoichiometric cell. (c) Atomic DOS showing thepstates of Oicompared withpstates for apical and planar oxygens in a stoichiometric cell. (d) Atomic DOS showing thedstates of the closest Y1 and Y2 to Oicompared with the average Ydstates in a stoichiometric cell. Figure 5: Electronic structure. ( a ) Total electronic density of states (DOS) for a perfect 120 atom YMnO 3 cell and a 121 atom cell of YMnO 3 with one O i (YMnO 3.04 ). ( b ) Atomic DOS showing the d states for Mn 3+ and Mn 4+ coordinating O i compared with Mn 3+ d states in a stoichiometric cell. ( c ) Atomic DOS showing the p states of O i compared with p states for apical and planar oxygens in a stoichiometric cell. ( d ) Atomic DOS showing the d states of the closest Y1 and Y2 to O i compared with the average Y d states in a stoichiometric cell. Full size image Functional properties We now address the impact of O i on the electronic properties. The introduction of O i between three Mn ( Fig. 3a ) gives three edge-sharing octahedra. As these octahedra are strongly distorted, the crystal field experienced by the d-electrons of Mn coordination O i does not change significantly compared with the trigonal bipyramidal crystal field in the perfect crystal. The most obvious change in electronic structure, in Fig. 5 , caused by O i is the appearance of a non-bonding defect state in the band gap mainly consisting of Mn 4+ states and O i 2 p x and 2 p y states. A fraction of the occupied Mn d states closest to the Fermi energy is lifted above E F on inclusion of O i as electron density is donated from Mn 3 d to O 2 p . The corresponding binding states are easily seen at the bottom of the valence band. Even though charge transfer is not complete, this can formally be regarded as the oxidation of Mn 3+ to Mn 4+ , creating holes in the valence band and p- type electronic conductivity. The p -DOS of interstitial oxygen is very similar to that of planar oxygen, which is also coordinated by only Mn, while it differs significantly from the p -DOS of apical oxygen, which is coordinated by both Mn and Y. The highly localized character of the defect state in the band gap is characteristic for the electronic structure of an acceptor doped material, and direct experimental detection of O i in low concentrations, by for example spectroscopic techniques, would be challenging. With increasing O i concentration, the defect state becomes less localized, as expected (See Supplementary Figure 9 for DOS and band structure of a 30 atom unit cell, YMnO 3.16 ). To address the impact of O i on the ferroelectric properties we calculated the spontaneous polarization ( P S ) by the Berry phase method to 7.8 μC cm −2 for the perfect structure, and 7.2 μC cm −2 after inclusion of one O i in a 120 atom supercell. A simple point charge model gave 7.8 and 7.0 μC cm −2 for stoichiometric YMnO 3 and oxidized YMnO 3.04 , respectively. Although the effect of O i on the spontaneous polarization is subtle, the charge compensating holes will raise the electrical conductivity and be detrimental to the macroscopic ferroelectric performance. However, in improper ferroelectrics like YMnO 3 , charged domain walls (DW) display anisotropic conductance due to the accumulation of mobile charge carriers [27] . Interstitial oxygen with formal charge −2 can screen the electrostatic field at head-to-head DWs, while charge compensating holes can screen tail-to-tail DW. Engineering point defect populations at DWs has great potential for tuning the properties of DWs as functional elements for electronics [28] , [29] , [30] , [31] . To summarize, we have shown that interstitial oxygen is the dominating point defect in YMnO 3 and the source of p -type electronic conductivity at ambient conditions. Interstitial oxygen is an enthalpy stabilized point defect, implying that YMnO 3 is not only metastable with respect to Y 2 O 3 and YMn 2 O 5 , in accordance with the phase diagram [32] , it is also metastable with respect to oxidation towards the limiting case of Y 3 Mn 3 O 10 . A bulk YMnO 3 sample will however not oxidize completely at ambient conditions for kinetic reasons; the diffusion length is too large compared with the relatively low ionic mobility at room temperature. However, at the nanoscale, in thin films and at surfaces, oxidation will occur spontaneously also at ambient conditions. This emphasizes the necessity and potential which lies in controlling the thermal and atmospheric history of hexagonal manganite materials in order to tailor the point defect population, charge carrier concentration and physical properties. Experimental Bulk YMnO 3 powder was prepared by firing pressed pellets of dried and mixed Y 2 O 3 and MnO 2 twice for 24 h at 1,300 °C in air. Porous polycrystalline bars with a density of 43% were sintered from phase pure YMnO 3 powder with 20 wt% carbon black as a pore filler for 2 h at 1,500 °C in air and scanning electron micrographs of the fracture surfaces of the porous bars are given in Supplementary Fig. 10 . Porous bars were used to increase the total surface area accessible to oxygen surface exchange. Four-point electrical conductivity measurements were performed on a porous polycrystalline bar in flowing O 2 and N 2 (ref. 33 ). Impedance spectroscopy measurements (Novotherm, Novocontrol Technologies) were conducted within a temperature range from 30 to 350 °C on disc shaped samples using frequencies between 1 Hz and 1 MHz. Before measurement the samples were annealed in flowing oxygen resp. nitrogen for 24 h at 350 °C. Thermogravimetry (TGA) was done with a Netzsch STA 449C Jupiter in flowing N 2 and O 2 on nanoparticles with d XRD =49±4 nm (ref. 17 ). Seebeck coefficients were measured at 200–500 °C in flowing O 2 and N 2 with a ProboStat setup (NorECs AS) on a porous bar in a vertical tubular furnace [34] . More details on the synthesis and characterization can be found in Supplementary Methods . Computational Density functional theory calculations were performed with the VASP [35] , [36] code and the spin polarized GGA+ U implementation of Dudarev [37] with the PBEsol functional [38] . A Hubbard U of 5 eV was applied to the Mn 3 d orbitals in order to reproduce the experimental band gap [39] and lattice parameters [40] . The projector augmented wave [41] method was used treating Y(4 s ,4 p ,4 d, 5 s ), Mn(3 s ,3 p ,3 d ,4 s ) and O(2 s ,2 p ) as valence electrons and a plane-wave cutoff energy of 550 eV. Brillouin zone integration was done on a Γ -centered 4 × 4 × 2 mesh for the 30 atom unit cell and with the number of k -points reduced accordingly for supercells. The non-collinear magnetic structure was approximated by a frustrated collinear antiferromagnetic (F-AFM) [42] order in most of the calculations, which does not give significantly different results from calculations with the true non-collinear magnetic order. Geometry optimization was done until the forces on the ions were below 0.005 eV Å −1 for 121 atom cells and 0.02 for 541 atom cells. The reducing and oxidizing limit for the chemical potential of oxygen varies from −7.1 to −1.9 eV. The defect formation energy of O i was 0.03 eV lower in a 121 atom cell than in a 541 atom cell (See Supplementary Fig. 11 ). Bader analysis [43] gave charges of +1.90 and +1.73 for Mn 4+ and Mn 3+ , respectively. For the nudged elastic band [44] (NEB) calculations we used five intermediate images for the O i migration path and a Hubbard U =5 eV was applied to reproduce the nature of the localized electron holes (comparison with U =0 eV can be found in the Supplementary Fig. 8b ). A frustrated antiferromagnetic (F-AFM) order was also used for the calculation of the energy barriers. Comparison between A-type AFM and F-AFM magnetic order is given in Supplementary Fig. 8c , and was set so that no spin flipping on the Mn ions occurred during the migration of O i in order to isolate the effect of pure migration. The ferroelectric polarization was calculated with the Berry phase method [45] . VESTA was used for visualizing structures [46] . Data availability The data that support the findings of this study are available from the authors on reasonable request. How to cite this article: Skjærvø, S. H. et al . Interstitial oxygen as a source of p -type conductivity in hexagonal manganites. Nat. Commun. 7, 13745 doi: 10.1038/ncomms13745 (2016). Publisher’s note : Springer Nature remains neutral with regard to jurisdictional claims in published maps and institutional affiliations.